A C–H bond activation-based catalytic approach to tetrasubstituted chiral allenes Enantioselective synthesis of fully substituted allenes has been a challenge due to the non-rigid nature of the axial chirality, which spreads over three carbon atoms. Here we show the commercially available simple Rh complex may catalyse the CMD (concerted metalation/deprotonation)-based reaction of the readily available arenes with sterically congested tertiary propargylic carbonates at ambient temperature affording fully substituted allenes. It is confirmed that the excellent designed regioselectivity for the C–C triple bond insertion is induced by the coordination of the carbonyl group in the directing carbonate group as well as the steric effect of the tertiary O-linked carbon atom. When an optically active carbonate was used, surprisingly high efficiency of chirality transfer was realized, affording fully substituted allenes in excellent enantiomeric excess (ee). Allenes have been becoming more and more important due to their presence in nature and the recent demonstration of their great potentials in modern organic chemistry with very nice reactivities, which led to their versatile applications in the efficient total syntheses of some natural products and drugs [1] , [2] , [3] , [4] . Thus, the highly selective synthesis of allenes is of great importance [5] , [6] , [7] , [8] , [9] , [10] . On the basis of recent advancements, the enantioselective synthesis of 1,3-disubstituted or 1,1,3-trisubstituted allenes has been at least partially solved [6] , however, enantioselective synthesis of tetrasubstituted is still a challenge [6] , [7] , [8] , [9] , [10] . Here we propose that the well-established CMD (concerted metalation/deprotonation) process of arenes [11] , [12] , [13] , [14] , [15] , [16] would generate organometallic intermediates in situ , which would, in principle, react with 2-alkynylic derivatives with an appropriate leaving group to afford allenes via regioselectivity-reversed insertion and thermodynamically non-favoured β-elimination ( Fig. 1b ). However, the challenge is the regioselectivity of the carbometalation of the C–C triple bond with the in situ generated aryl metallic species [17] , [18] , [19] , [20] , [21] , [22] since the reported insertion reaction with the C–C triple bond in propargylic alcohols affording the [4+2]-products with the undesired regioselectivity [18] . To achieve our goal, we proposed to reverse the regioselectivity by installing a directing entity in the propargylic leaving group, thus avoiding the formation of undesired B -type insertion intermediate [18] . In addition, it should be noted that stereospecific β-elimination of the targeted intermediate A providing highly optically active allenes is challenging as the Rh-catalysed reaction of stoichiometric amount each of aryl boronic acids and optically active propargylic acetates with forming allenes in an extremely low efficiency of chirality transfer due to the mixed syn- and anti-non-stereospecific β-elimination [23] , [24] , [25] . In such a well-designed process, the oxidation state of the metal in the catalyst would remain the same, thus, making it catalytic in [M] and free of any oxidants for the regeneration of catalyst in many of C–H functionalization reactions [11] , [12] , [13] , [14] , [15] , [16] . 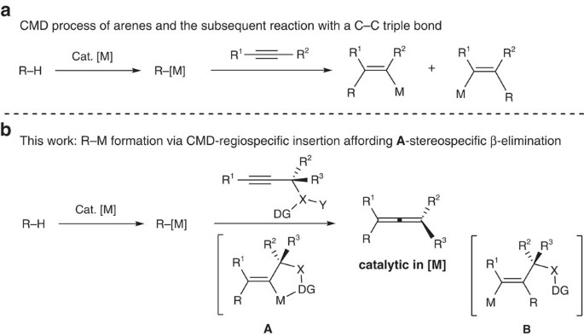Figure 1: Carbometallations of alkynes. (a) CMD-based reaction of R–H with alkynes. (b) This work: new concept and challenge for allene synthesis. Figure 1: Carbometallations of alkynes. ( a ) CMD-based reaction of R–H with alkynes. ( b ) This work: new concept and challenge for allene synthesis. Full size image Herein, we wish to report the realization of such a concept for the synthesis of tetrasubstituted allenes via the commercially available [Cp*RhCl 2 ] 2 catalysed coupling between readily available essential chemicals, that is, arenes and 2-alkynylic carbonates with a surprisingly high efficiency for point-to-axial chirality transfer. After careful studies, it is believed that the directing group and the steric effect of the tertiary 2-alkynylic carbonates are responsible for the reversed regioselectivity for the insertion of the C–C triple bond. Identification of the leaving group With the purpose of synthesizing the most challenging tetra-subtituted allenes, we first tried to identify a proper leaving group for the tertiary propargylic alcohol ( Fig. 2 ): When N -methoxybenzamide 1a was reacted with tertiary propargylic methyl ether 2a 1 in a mixed solvent of MeOH and water (20/1) under the catalysis of [Cp*RhCl 2 ] 2 at room temperature, no allene was formed with 1a being recovered; when we introduced a phosphate as leaving group ( 2a 2 ), interestingly the expected tetrasubstituted allene 3aa was afforded in 8% NMR yield! [18] When propargylic acetate 2a 3 was used, the yield was improved to 46%; with these results in hand, we envisioned to have a methoxy group to replace the methyl group in the acetyl unit to increase the electron density of the carbonyl oxygen, that is, carbonate: to our delight, the carbonate 2a was indeed the best and the yield was further improved to 76%. After further optimization of the parameters of the reaction, the reaction of 1.2 equiv. 1a and 2a in a mixed solvent of MeOH and water (20/1) under the catalysis of [Cp*RhCl 2 ] 2 with 30 mol% NaOAc as base was chosen as the optimized reaction conditions for further study (for details of optimization, see Supplementary Table 1 ). 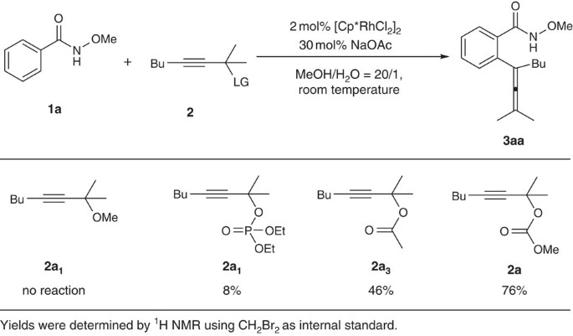Figure 2: The effect of leaving groups. A carbonate was found to be the most efficient. Figure 2: The effect of leaving groups. A carbonate was found to be the most efficient. Full size image Substrate scope The reaction proceeded well on a gram scale, affording 3aa in 82% yield ( Fig. 3 ). Having the optimized reaction conditions in hand, the generality of the reaction was then investigated. Electron-donating groups such as t -butyl and methoxy as well as electron-withdrawing groups such as CF 3 and F in the aryl unit were all tolerated in the amides giving the corresponding fully substituted allenes in good to excellent yields ( Fig. 3 ; 3aa , 3ba , 3ca , 3da , 3ea , 3bf and 3cf ). It was noteworthy that when a meta-substituted 1d was used, the less hindered C–H bond was exclusively functionalized and an o -fluorine atom did not hamper the reaction affording 3ea in 79% yield ( Fig. 3 , 3da and 3ea ). The R 1 , R 2 , and R 3 groups in the 2-alkynylic carbonate could be alkyl or aryl groups ( Fig. 3 ; 3ac , 3ad , 3ae , 3af , 3ag , 3ah , 3bf and 3cf ). Substrates with sterically hindered i -Bu or o -tolyl groups also worked ( Fig. 3 , 3ac and 3ag ). 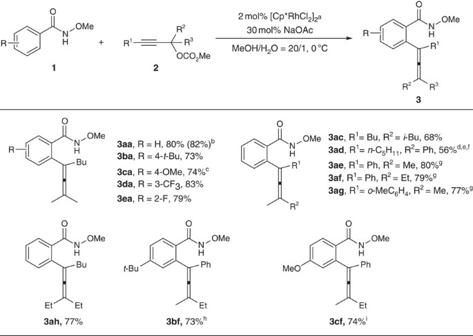Figure 3: Substrate scope. Electron-withdrawing and electron-donating as well as bulky groups were all tolerated.aThe reaction was conducted with1(1.2 mmol),2(1 mmol), [Cp*RhCl2]2(0.02 mmol), NaOAc (0.3 mmol), MeOH (6 ml), and H2O (0.3 ml) and monitored by TLC.bReaction was conducted on 7 mmol scale.cReaction was conducted at −10 °C,1a(1.3 mmol) and NaOAc (1 mmol) was used.dReaction was conducted at room temperature.e1a(2 mmol), [Cp*RhCl2]2(0.05 mmol) was used.fThe acetate was used instead because of the unstability of the carbonate.g1a(1.5 mmol), [Cp*RhCl2]2(0.04 mmol) was used.h1b(1.5 mmol), [Cp*RhCl2]2(0.04 mmol) was used.i1c(1.5 mmol), [Cp*RhCl2]2(0.04 mmol) was used. Figure 3: Substrate scope. Electron-withdrawing and electron-donating as well as bulky groups were all tolerated. a The reaction was conducted with 1 (1.2 mmol), 2 (1 mmol), [Cp*RhCl 2 ] 2 (0.02 mmol), NaOAc (0.3 mmol), MeOH (6 ml), and H 2 O (0.3 ml) and monitored by TLC. b Reaction was conducted on 7 mmol scale. c Reaction was conducted at −10 °C, 1a (1.3 mmol) and NaOAc (1 mmol) was used. d Reaction was conducted at room temperature. e 1a (2 mmol), [Cp*RhCl 2 ] 2 (0.05 mmol) was used. f The acetate was used instead because of the unstability of the carbonate. g 1a (1.5 mmol), [Cp*RhCl 2 ] 2 (0.04 mmol) was used. h 1b (1.5 mmol), [Cp*RhCl 2 ] 2 (0.04 mmol) was used. i 1c (1.5 mmol), [Cp*RhCl 2 ] 2 (0.04 mmol) was used. Full size image Compatibility of functional groups To show the robustness of our newly developed catalytic allene synthesis strategy, substrates with synthetically useful yet sensitive functional groups were explored without any protection: to our delight, Cl, Br, CO 2 Me, CN and even unprotected free alcohol were all well tolerated, showing the broad synthetically attractive functional group compatibility ( Fig. 4 ; 3fa , 3ff , 3ga , 3hi , 3ij and 3al ). The structure of 3fa was further confirmed by X-ray diffraction study. (For details of the X-ray diffraction study of 3fa , see Supplementary Dataset 1 and pages 96–97 in the Supplementary File .) Interestingly, even γ -(1-alkynyl)- γ -lactone 2m may be used to afford tetrasubstituted γ -allenoic acid 3am directly in an atom-economic way ( Fig. 4 ; 3am ). 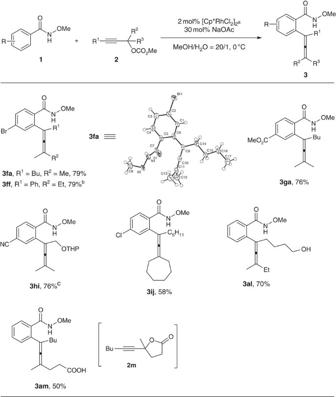Figure 4: Functional group compatibility. Many synthetically useful yet sensitive functional groups survived without any protection.aThe reaction was conducted with1(1.2 mmol),2(1 mmol), [Cp*RhCl2]2(0.02 mmol), NaOAc (0.3 mmol), MeOH (6 ml) and H2O (0.3 ml) and monitored by TLC.b1f(1.5 mmol), [Cp*RhCl2]2(0.04 mmol) was used.c[Cp*RhCl2]2(0.04 mmol) was used. Figure 4: Functional group compatibility. Many synthetically useful yet sensitive functional groups survived without any protection. a The reaction was conducted with 1 (1.2 mmol), 2 (1 mmol), [Cp*RhCl 2 ] 2 (0.02 mmol), NaOAc (0.3 mmol), MeOH (6 ml) and H 2 O (0.3 ml) and monitored by TLC. b 1f (1.5 mmol), [Cp*RhCl 2 ] 2 (0.04 mmol) was used. c [Cp*RhCl 2 ] 2 (0.04 mmol) was used. Full size image Regioselectivity The regioselectivity is an important issue when >1 C–H bonds could be activated. When N -methoxy-2-naphthylcarboxylic amide 1j was used to react with 2a , the less hindered C–H bond was exclusively functionalized affording 3ja ( Fig. 5 , equation (a)). A heteroaryl N -methoxyamide 1k was also a suitable substrate and C–H bond in the thiene moiety was exclusively functionalized giving 3ka in 81% yield ( Fig. 5 , equation (b); also see: Fig. 3 ; 3da ). 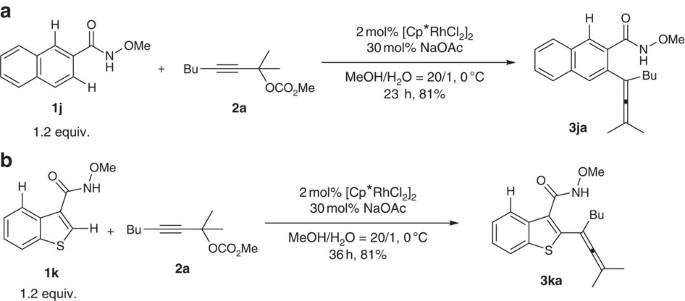Figure 5: Regioselectivity of the reaction. (a) The less hindered C–H bond was exclusively functionalized. (b) The thiophene C–H bond was exclusively functionalized. Figure 5: Regioselectivity of the reaction. ( a ) The less hindered C–H bond was exclusively functionalized. ( b ) The thiophene C–H bond was exclusively functionalized. Full size image Other directing groups With this protocol in hand, we reasoned that such a concept should be working also with directing groups other than the N -methoxy amide. In fact, arenes 1l and 1m with directing groups of pyridine and pyrazole could also react with 2a forming tetrasubstituted allenes 3la and 3ma . Thus, such a protocol may be applied to other type of substrates with functionalizable C–H bonds ( Fig. 6 ). 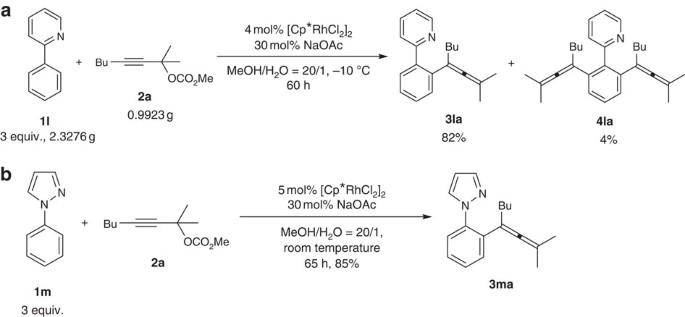Figure 6: The scope of directing groups. Pyridine and pyrazole could also be suitable directing groups. Figure 6: The scope of directing groups. Pyridine and pyrazole could also be suitable directing groups. Full size image Synthetic applications The synthetic applications for the formed products were also conducted: 3la could react with an extra propargyl carbonate, affording bis-allene 5 , which showed the possibility of a stepwise allenylation ( Fig. 7 , equation (a)). The N -methoxyamide moiety in 3aa could direct a well-known [4+2] addition with 1,2-diphenylethyne giving isoquinolinone 6 with allene intact ( Fig. 7 , equation (b)) [18] . 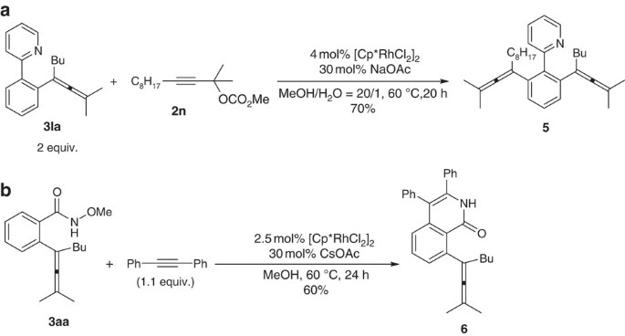Figure 7: The synthetic applications. (a) A stepwise allenylation. (b) A [4+2] addition affording isoquinolinone. Figure 7: The synthetic applications. ( a ) A stepwise allenylation. ( b ) A [4+2] addition affording isoquinolinone. Full size image In order to further study the mechanism, following experiments have been conducted. Firstly, N -methoxy-2-naphthamide 1j was treated with 20 mol% of [Cp*RhCl 2 ] 2 to in situ generate the naphthyl Rh species, its reaction with secondary propargylic carbonate 2o demonstrated the opposite regioselectivity, leading to the undesired reported B -type insertion regioisomer exclusively [18] , finally yielding the [4+2] product 7 observed by Fagnou, Glorius, Rovis, Cramer and other groups ( Fig. 8 ; for details of the X-ray diffraction study of 7 , see Supplementary Dataset 2 and page 108 in the Supplementary File ) [17] , [18] , [19] , [20] , [21] , [22] : the desired A -type insertion regioisomer, which would have led to the formation of allene via β-elimination, was not formed! Thus, we reasoned that there is a striking tertiary carbon atom effect here: in order to have the carbonyl group acts the directing group in this linear C–C triple bond environment, the tertiary carbon atom in the carbonate may push the carbonyl group for its easier coordination with Rh while having a weaker interaction with the to-be-inserted C–C triple bond. 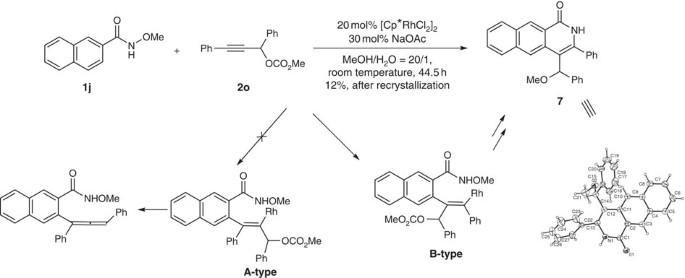Figure 8: Striking tertiary carbon atom effect. Secondary propargylic carbonate2oonly demonstrated the opposite regioselectivity. Figure 8: Striking tertiary carbon atom effect. Secondary propargylic carbonate 2o only demonstrated the opposite regioselectivity. Full size image In the second place, to our delight, when chiral carbonate S -2f (98% ee) was applied, axial chiral allenes were formed with an excellent ee (98% ee) with a surprisingly high efficiency of chirality transfer ( Fig. 9 ). The absolute configuration of chiral 3af was determined as S by X-ray diffraction study and the absolute configurations of other chiral allenes S -3bf , S -3cf and S -3ff were defined by analogy. (For details of the X-ray diffraction study of S -3af , see Supplementary Dataset 3 and page 110 in the Supplementary File .) These results further excluded the possibility of oxidative addition of propargylic carbonate with Rh to form allenyl rhodium intermediate (leading to racemization) [24] , [26] , [27] , which would react with arene via a CMD process followed by reductive elimination to afford the allene. 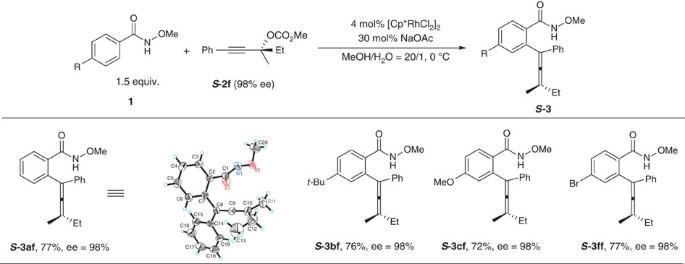Figure 9: Highly entioselective synthesis of tetra-substituted allenes by chirality transfer. Excellent efficiency of chirality transfer was found when using chiral carbonateS-2f. The reaction was conducted with1(0.3 mmol),2(0.2 mmol), [Cp*RhCl2]2(0.008 mmol), NaOAc (0.06 mmol), MeOH (1.2 ml), and H2O (0.06 ml) and monitored by TLC. The ees were determined by HPLC. Figure 9: Highly entioselective synthesis of tetra-substituted allenes by chirality transfer. Excellent efficiency of chirality transfer was found when using chiral carbonate S -2f . The reaction was conducted with 1 (0.3 mmol), 2 (0.2 mmol), [Cp*RhCl 2 ] 2 (0.008 mmol), NaOAc (0.06 mmol), MeOH (1.2 ml), and H 2 O (0.06 ml) and monitored by TLC. The ees were determined by HPLC. Full size image The kinetic isotope effect was measured by parallel experiments of 1a and 1a-D 5 with 2a . The kinetic isotope effect value of 2.1 demonstrated that C–H activation should be the rate-determining step ( Fig. 10a ) [28] . 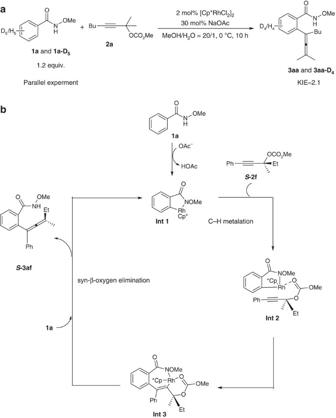Figure 10: Mechanistic issues (a) The kinetic isotope effect. A kinetic isotope effect value of 2.1 was measured. (b) Plausible mechanism. The carbonate carbonyl and tertiary carbon atom effect accounts for the reversed regioselectivity and the excellent efficiency of chirality was realized via syn-β-elimination. Figure 10: Mechanistic issues ( a ) The kinetic isotope effect. A kinetic isotope effect value of 2.1 was measured. ( b ) Plausible mechanism. The carbonate carbonyl and tertiary carbon atom effect accounts for the reversed regioselectivity and the excellent efficiency of chirality was realized via syn-β-elimination. Full size image According to these results, a plausible mechanism has been proposed as shown in Fig. 10b . The first step of the rate-determining CMD of arenes would form rhodabicyclic intermediate Int 1 (ref. 29 ), which is followed by coordination with the carbonyl oxygen of the carbonate forming Int 2 . Subsequent ‘reversed’ regiospecific insertion of the alkyne moiety [18] directed by the carbonyl group in propargyl carbonate S -2f afforded with the carbonyl oxygen-coordinated rhoda-tricyclic Int 3 (refs 11 , 12 , 13 , 14 ). The steric effect may set the carbonyl group for its better coordination with Rh and the subsequent defined coordination/insertion with C–C triple bond leading to the formation of Int 3- type tricyclic intermediate, which directly underwent syn-β-oxygen elimination to form the final product S -3af and relieves the catalytically active Rh(III) species [30] , [31] , [32] , [33] , [34] , [35] , [36] , [37] . It should be noted that usually anti-β-oxygen elimination was observed [23] , [24] , [25] . This syn-β-oxygen elimination explains the excellent efficiency for chirality transfer since it was reported that the Rh-catalysed reaction of optically active propargylic acetates with aryl boronic acids forming allenes in an extremely low efficiency of chirality transfer [23] , [24] , [25] . In conclusion, a completely new protocol has been established for the efficient synthesis of allenes using the readily available arenes and 2-alkynylic carbonates as the starting materials at room temperature with very good yields. The reaction is compatible with ambient air, moisture and a broad array of synthetically useful functional groups such as Cl, Br, CO 2 Me, CN, free alcohol and even acid. The formed tetrasubstituted allenes could be transformed to isoquinolinone as while as bis-allene products. In fact, in some cases, very minor amount of cycloisomerisation products were observed in the NMR analysis of the crude products. Excellent selectivity for alkyne insertion must be induced by combination of carbonyl directing group as well as the steric effect of tertiary carbon centre. The surprisingly high efficiency of chirality transfer addresses the challenge for the synthesis of not-readily available highly optically active fully substituted allenes from a highly optically active carbonate. This protocol for the synthesis of allenes will trigger such reactions using other types of substrates with functionalizable C–H bonds and propargylic alcohol derivatives, thus, will be of high interest in organic chemistry and related disciplines. Further studies in this area are being pursued in our laboratory. Materials [Cp*RhCl 2 ] 2 was purchased from Strem Chemicals. N -methoxybenzamides [22] and known propargylic carbonates [38] were prepared according to the literature procedures. Other commercially available chemicals were purchased and used without additional purification unless noted otherwise. General spectroscopic methods 1 H NMR spectra were recorded on a Bruker-300 MHz spectrometer and 13 C NMR spectra were recorded at 75 MHz. All 1 H NMR experiments were measured with tetramethylsilane (0 p.p.m.) or the signal of residual CHCl 3 (7.26 p.p.m.) in CDCl 3 as the internal reference, 13 C NMR experiments were measured in relative to the signal of CDCl 3 (77.0 p.p.m. ), and 19 F NMR experiments were measured in relative to the signal of residual CFCl 3 (0 p.p.m.) in CDCl 3 . Infrared spectra were recorded from this films of pure samples on sodium chloride plates for liquid or in the form of KBr discs for the solid samples. Mass and high-resolution mass spectrometry (HRMS) spectra were carried out in Electron Ionization (EI) mode. Thin-layer chromatography (TLC) was performed on pre-coated glass-back plates and visualized with ultraviolet light at 254 nm. Flash column chromatography was performed on silica gel. 1 H NMR, 13 C NMR and High Performance Liquid Chromatography (HPLC) spectra (for chiral compounds) are supplied for all compounds: see Supplementary Figs 1–82 . See Supplementary Methods for the characterization data of compounds not listed in this part. Synthesis of 3aa To a dried Schlenk tube equipped with a Teflon-coated magnetic stirring bar were added N -methoxybenzamide 1a (182.1 mg, 1.2 mmol), [Cp*RhCl 2 ] 2 (12.6 mg, 0.02 mmol), NaOAc (24.3 mg, 0.3 mmol), methyl (2-methyloct-3-yn-2-yl) carbonate 2a (198.5 mg, 1 mmol), MeOH (6 ml), and H 2 O (0.3 ml) sequentially at room temperature. After being stirred for 19 h at 0 °C, the reaction was complete as monitored by TLC. Filtration through a short column of silica gel (eluent: ethyl acetate 20 ml × 3) and evaporation afforded the crude product, which was purified by flash column chromatography on silica gel (eluent: petroleum/ethyl acetate/dichloromethane=10/1/0.1/ to 5/1/0.5) to afford 3aa (218.6 mg, 80%): solid; melting point (m.p.) 66.9–68.1 °C (hexane/ethyl acetate); 1 H NMR (300 MHz, CDCl 3 ) δ 8.74 (brs, 1 H, NH), 7.58 (d, J =7.2 Hz, 1 H, Ar–H), 7.39 (td, J 1 =7.5 Hz, J 2 =1.3 Hz, 1 H, Ar–H), 7.32–7.21 (m, 2 H, Ar–H), 3.86 (s, 3 H, OCH 3 ), 2.29 (t, J =7.1 Hz, 2 H, CH 2 ), 1.76 (s, 6 H, 2 × CH 3 ), 1.49–1.27 (m, 4 H, 2 × CH 2 ), 0.89 (t, J =6.9 Hz, 3 H, CH 3 ); 13 C NMR (75 MHz, CDCl 3 ) δ 201.3, 167.9, 138.3, 131.5, 130.5, 129.1, 126.7, 102.9, 97.6, 64.3, 33.6, 30.0, 22.1, 20.3, 13.9; IR (neat, cm −1 ) 3,188, 2,956, 2,931, 2,875, 2,859, 1,953, 1,659, 1,590, 1,495, 1,465, 1,440, 1,299, 1,156, 1,035; MS (EI, 70 eV) m / z (%) 273 (M + , 4.18), 242 (100); Anal. Calcd for C 17 H 23 NO 2 : C 74.69, H 8.48, N 5.12. Found: C 74.89, H 8.62, N 4.89. Synthesis of 5 To a dried Schlenk tube equipped with a Teflon-coated magnetic stirring bar were added [Cp*RhCl 2 ] 2 (12.5 mg, 0.02 mmol), NaOAc (12.8 mg, 0.15 mmol), 3la (277.5 mg, 1.0 mmol), 2n (126.8 mg, 0.5 mmol), MeOH (3 ml), and H 2 O (0.15 ml) sequentially at room temperature. The Schlenk tube was then equipped with a condenser. After being stirred for 20 h at 60 °C, the reaction was complete as monitored by TLC (eluent: petroleum ether/ethyl acetate=20/1). Filtration through a short column of silica gel (eluent: ethyl acetate 20 ml × 3) and evaporation afforded the crude product, which was purified by flash column chromatography on silica gel (eluent: hexane/ethyl acetate=100/1) to afford 5 (158.4 mg, 70%): oil; 1 H NMR (300 MHz, CDCl 3 ) δ 8.61 (d, J =4.2 Hz, 1 H, Ar–H), 7.62 (td, J 1 =7.8 Hz, J 2 =1.8 Hz, 1 H, Ar–H), 7.30–7.22 (m, 2 H, Ar–H), 7.21–7.11 (m, 3 H, Ar–H), 2.01–1.90 (m, 4 H, CH 2 × 2), 1.39 (s, 12 H, CH 3 × 4), 1.32–1.10 (m, 16 H, CH 2 × 8), 0.87 (t, J =6.8 Hz, 3 H, CH 3 ), 0.80 (t, J =7.1 Hz, 3 H, CH 3 ); 13 C NMR (75 MHz, CDCl 3 ) δ 201.2, 160.0, 148.6, 139.92, 139.89, 138.1, 134.9, 127.5, 127.4, 125.9, 121.1, 103.3, 103.2, 95.6, 34.2, 33.9, 31.8, 29.8, 29.5, 29.3, 29.0, 27.6, 22.6, 22.1, 20.4, 14.1, 14.0; IR (neat, cm −1 ) 3,059, 2,955, 2,926, 2,854, 1,962, 1,932, 1,588, 1,571, 1,561, 1,452, 1,419, 1,377, 1,361, 1,188, 1,023; MS (EI, 70 eV) m / z (%) 455 (M + , 18.96), 84 (100); HRMS Calcd for C 33 H 45 N (M + ): 455.3552. Found: 455.3553. Synthesis of 6 To a dried Schlenk tube equipped with a Teflon-coated magnetic stirring bar were added 3aa (109.3 mg, 0.4 mmol), 1,2-diphenylethyne (78.6 mg, 0.44 mmol), [Cp*RhCl 2 ] 2 (6.2 mg, 0.01 mmol), CsOAc (22.4 mg, 0.12 mmol), and MeOH (2 ml) sequentially at room temperature. The Schlenk tube was then equipped with a condenser. After being stirred for 24 h at 60 °C, the reaction was complete as monitored by TLC (eluent: petroleum ether/ethyl acetate=3/1). Filtration through a short column of silica gel (eluent: (dichloromethane/ethyl acetate=1/1) (20 ml × 3)) and evaporation afforded the crude product, which was purified by flash column chromatography on silica gel (eluent: dichloromethane/ethyl acetate=20/1) to afford 6 (101.1 mg, 60%): solid; m.p. 199.0–200.4 °C (hexane/ethyl acetate); 1 H NMR (300 MHz, CDCl 3 ) δ 9.02 (s, 1 H, Ar–H), 7.44 (t, J =7.8 Hz, 1 H, Ar–H), 7.34–7.10 (m, 12 H, Ar–H), 2.33 (t, J =7.1 Hz, 2 H, CH 2 ), 1.76 (s, 6 H, CH 3 × 2), 1.53–1.29 (m, 4 H, CH 2 × 2), 0.90 (t, J =7.1 Hz, 3 H, CH 3 ); 13 C NMR (75 MHz, CDCl 3 ) δ 199.0, 161.6, 142.7, 140.2, 137.2, 136.4, 135.1, 131.9, 131.7, 129.8, 129.0, 128.5, 128.3, 127.1, 124.9, 122.5, 116.8, 106.9, 95.6, 34.7, 30.5, 22.5, 20.9, 14.2; IR (neat, cm −1 ) 3,453, 3,165, 3,027, 2,947, 2,929, 2,869, 2,849, 1,947, 1,642, 1,596, 1,584, 1,486, 1,462, 1,441, 1,311, 1,144; MS (EI, 70 eV) m / z (%) 419 (M + , 31.3), 376 (100); HRMS Calcd for C 30 H 29 NO (M + ): 419.2249. Found: 419.2247. Anal. Calcd for C 30 H 29 NO: C 85.88, H 6.97, N 3.34. Found: C 84.90, H 6.96, N 3.31. Synthesis of 7 Following procedure for the synthesis of 3aa , the reaction of 1j (303.1 mg, 1.5 mmol), [Cp*RhCl 2 ] 2 (185.5 mg, 0.3 mmol), NaOAc (36.9 mg, 0.45 mmol), 2o (400.1 mg, 1.5 mmol), MeOH (9 ml), and H 2 O (0.45 ml) at room temperature afforded impure 7 with impurities (136.8 mg) (eluent: Hexane/ethyl acetate/dichloromethane=10/1/0.2 to 8/1/0.5), which was further purified by recrystallization (hexane/THF) afford pure 7 (69.7 mg, 12%): solid; m.p. 117.5–119.0 °C (hexane/THF); 1 H NMR (300 MHz, CDCl 3 ) δ 9.02 (s, 1 H, Ar–H), 8.91 (bs, 1 H, NH), 8.32 (s, 1 H, Ar–H), 8.06–7.94 (m, 1 H, Ar–H), 7.75–7.66 (m, 1 H, Ar–H), 7.55–7.40 (m, 8 H, Ar–H), 7.36–7.17 (m, 4 H, Ar–H), 5.57 (s, 1 H, CH), 3.31 (s, 3 H, CH 3 ); 13 C NMR (75 MHz, CDCl 3 ) δ 163.2, 141.6, 139.4, 135.1, 134.8, 131.2, 131.1, 129.6, 129.04, 128.97, 128.81, 128.77, 128.5, 128.3, 127.8, 127.1, 126.6, 126.2, 124.5, 111.1, 80.3, 56.5; IR (neat, cm −1 ) 3,181, 3,057, 3,027, 2,927, 2,890, 2,819, 1,659, 1,625, 1,600, 1,493, 1,448, 1,355, 1,312, 1,089, 1022; MS (EI, 70 eV) m/z (%) 392 (M + +1, 30.89), 391 (M + , 100); HRMS Calcd for C 27 H 21 NO 2 (M + ): 391.1572. Found: 391.1571. Synthesis of S -3af Following procedure for the synthesis of 3aa , the reaction of 1a (45.6 mg, 0.3 mmol), [Cp*RhCl 2 ] 2 (4.8 mg, 0.008 mmol), NaOAc (5.3 mg, 0.06 mmol), S -2f (98% ee, 45.9 mg, 0.2 mmol), MeOH (1.2 ml), and H 2 O (0.06 ml) at 0 °C afforded S -3af (46.6 mg, 77%) (eluent: petroleum/ethyl acetate/dichloromethane=5/1/0.5): 98% ee (HPLC conditions: Chiralcel AD-H column, hexane/ i -PrOH=10/1, 1.0 ml min −1 , λ =207 nm, t R(minor) =21.9 min, t R(major) =24.5 min); solid; m.p. 99.9–101.1 °C (hexane/ethyl acetate); 1 H NMR (300 MHz, CDCl 3 ) δ 8.66 (s, 1 H, NH), 7.78 (d, J =7.5 Hz, 1 H, Ar–H), 7.53–7.14 (m, 8 H, Ar–H), 3.45 (s, 3 H, OCH 3 ), 2.27–2.06 (m, 2 H, CH 2 ), 1.90 (s, 3 H, CH 3 ), 1.13 (t, J =7.4 Hz, 3 H, CH 3 ); 13 C NMR (75 MHz, CDCl 3 ) δ 202.0, 166.6, 137.2, 135.6, 132.5, 131.20, 131.18, 129.6, 128.6, 127.9, 127.1, 126.5, 107.5, 106.5, 63.9, 27.4, 18.7, 12.3; IR (neat, cm −1 ) 3,199, 3,058, 3,018, 2,966, 2,932, 1,947, 1,659, 1,595, 1,491, 1,456, 1,439, 1,310, 1,159, 1,031; MS (EI, 70 eV) m / z (%) 307 (M + , 1.69), 246 (100); Anal. Calcd for C 20 H 21 NO 2 : C 78.15, H 6.89, N 4.56. Found: C 77.98, H 6.88, N 4.34. How to cite this article: Shangze, W. et al . A C–H bond activation-based catalytic approach to tetrasubstituted chiral allenes. Nat. Commun. 6:7946 doi: 10.1038/ncomms8946 (2015).